Vibrationally induced inversion of photoelectron forward-backward asymmetry in chiral molecule photoionization by circularly polarized light Electron–nuclei coupling accompanying excitation and relaxation processes is a fascinating phenomenon in molecular dynamics. A striking and unexpected example of such coupling is presented here in the context of photoelectron circular dichroism measurements on randomly oriented, chiral methyloxirane molecules, unaffected by any continuum resonance. Here, we report that the forward-backward asymmetry in the electron angular distribution, with respect to the photon axis, which is associated with photoelectron circular dichroism can surprisingly reverse direction according to the ion vibrational mode excited. This vibrational dependence represents a clear breakdown of the usual Franck–Condon assumption, ascribed to the enhanced sensitivity of photoelectron circular dichroism (compared with other observables like cross-sections or the conventional anisotropy parameter-β) to the scattering phase off the chiral molecular potential, inducing a dependence on the nuclear geometry sampled in the photoionization process. Important consequences for the interpretation of such dichroism measurements within analytical contexts are discussed. Photoelectron circular dichroism (PECD) has been applied for a decade as a direct chiroptical probe of gas-phase chiral systems and leads to astonishingly large asymmetries in the angular distribution of photoemitted electrons [1] . Because of this, PECD has been invoked as a symmetry-breaking mechanism that may be involved in the origin of life’s homochirality [1] , [2] . Such measurements may, however, also have analytical applications in the laboratory, a prospect recently enhanced by the demonstration of laser-based multiphoton PECD [3] . A fundamental aspect of PECD lies in its sensitivity to molecular structure, both static and dynamic, and here we consider more precisely vibrational dynamics in molecular photoionization. The coupling of electronic and nuclear motions is a striking manifestation of the complex many-particle dynamics involved in off-equilibrium systems, like excited molecules [4] . Such a coupling may be revealed, in the case of molecular electronic transitions, by the breakdown of the so-called Franck–Condon (FC) approximation. This approximation is widely accepted, as is its assumption of vertical transitions under the Born–Oppenheimer approximation (separation of the nuclear and electronic motions in view of their very different masses). Less commonly remarked, perhaps, is a secondary FC assumption that the transition matrix elements governing the probability of a given electronic transition do not depend on the nuclear geometry sampled during vibrational motion. Consequently, there can be an expectation of fully decoupled electron-nuclear dynamics. In the case of molecular photoionization, this means that the electron continuum features should be decoupled from the vibrational energy content of the cation so that, for instance, vibrational branching ratios measured in a photoelectron spectrum (PES) should be independent of the photon energy. Similarly, at a given energy, the electron angular distribution anisotropy parameters should be the same for all vibrational mode or quanta. Departures from this picture are of course encountered, most usually attributed to shape resonances in the continuum. These are known to be very sensitive to the nuclear geometries and have been mostly studied in diatomic [5] , [6] , [7] , and triatomic systems for which mode-specific [8] and symmetry-forbidden [9] effects have been reported. Recently, Jahnke et al . [10] reported a vibrational dependence in the molecular frame photoelectron angular distributions (MF-PADs) observed from C (1 s −1 ) photoionization of fixed-in-space CO molecules by circularly polarized light (CPL), at photon energies well removed from any shape resonance. These measurements also demonstrate the high sensitivity of MF-PADs to photoelectron scattering by the molecular potential and especially to the relative phases of the outgoing waves. Such invaluable information capable of yielding insight on vibrational dynamics is, in general, lost in the averaging owing to the random orientation in the laboratory frame, although with larger molecules molecule-frame measurements may anyway be unachievable. In this context, chiral molecule systems can offer an enhanced opportunity for investigating molecular photoionization, including vibrational dynamics, in great detail, even for randomly oriented samples, as we will demonstrate here. In such chiral systems, the laboratory frame PADs produced by photoionization with CPL can present a strong forward-backward asymmetry with respect to the light axis [11] . Although this was experimentally evidenced for the first time a decade ago [1] , the theoretical prediction of a PECD effect, by Ritchie [12] , further predates this by several decades. Ritchie [12] was able to show how a chiral asymmetry that arises in the pure electric dipole approximation can survive averaging over random molecular orientation, in effect because CPL defines a direction in space, with respect to which the different atoms of a given molecular enantiomer will be seen always in the same configuration by the incoming photon. Unlike conventional CD, PECD asymmetry is observed via a differential measurement, and may reach several tens of percentage [13] , [14] . Quantitatively, the PECD asymmetry equals 2 b 1 , where b 1 , the so-called dichroic parameter, is the coefficient of the odd first Legendre polynomial P 1 term in the angular distribution function , with θ being the angle between the direction of the emitted electron and the photon propagation axis and p the polarization of the ionizing radiation; p =0 for linear, p =+1 for left circular polarization (LCP), and p =−1 for right circular polarization (RCP). As symmetry considerations dictate that b 1 is non-zero only for chiral systems photoionized with CPL, it encapsulates the chiral contribution. Its origin lies in quantum interference terms between outgoing waves developed, as the photoelectron is scattered off the chiral molecular potential. More specifically, the interferences contributing to depend fully on the (odd) sine function of the relative phase between outgoing partial waves with adjacent angular momentum, ℓ and ℓ ±1 (refs 11 , 15 ). The parameters are therefore a much more sensitive probe of photoionization dynamics than both the regular anisotropy parameter, (containing a limited phase information, and that then depends on the even cosine function) and especially the cross-section, σ (which contains no phase information). Consequently, b 1 measurements can be used to probe molecular geometry and structures [16] , including conformers [17] , [18] , [19] , [20] and chemical substitution [21] . PECD seems, therefore, as an ideal tool to study also the dynamic interplay between electronic and nuclear motions upon photoionization. In this article, we report on a striking inversion of the chiral asymmetry according to the excited vibrational mode in the resulting cation, as observed by vibrationally resolved PECD, a clear breakdown of the FC approximation in molecular photoionization. The context So far, all published PECD studies have been vibrationally unresolved, except for a study of methyloxirane [22] performed at the single-photon energy of 22 eV, that is, about 12 eV above the ionization potential (IP), and that shows some weak modulations of the dichroism seemingly correlated with the partially resolved vibrational envelope of the highest occupied molecular orbital (HOMO). We decided to reinvestigate this showcase chiral molecular system but with much slower photoelectrons, that is, in the first eV above the IP where we expect PECD to be able to provide rich information on vibrational dynamics and for which our electron imaging technique is very efficient and capable of a high absolute energy resolution. Threshold photoelectron spectrum A threshold photoelectron spectrum (TPES) of methyloxirane in the HOMO region is presented in Fig. 1 , together with a vibrational simulation (using unscaled B3LYP/cc-pVTZ calculated harmonic frequencies). Although it is well known that TPES often departs from the direct ionization FC framework, the simulated intensities are obtained as FC factors, and the good semi-quantitative agreement allows the principal structure to be identified. The first intense peak ‘a’ is readily assigned to the origin (0-0) band whose intensity indicates rather similar ion and neutral geometries, consistent with the fact that the HOMO −1 ionization channel corresponds to the removal of a non-bonding electron from the O lone pairs. From this band, the adiabatic IP is determined at 10.25±0.01 eV. Other assignments made at low energy are single quantum excitations from the vibrationless neutral to normal modes of the cation corresponding to low-frequency skeletal deformation as follows: peak ‘b’ O-C 2 stretch plus methyl group wag; peak ‘c’ C-C-O scissoring (antisymmetric ring deformation); ‘d’ C-O-C symmetric bending (with accompanying CH 3 wag). Above 10.35 eV, peaks are mainly attributed to combination bands between several normal modes, out of the 24 allowed modes, but with ‘e’ and ‘f’ being single quantum CH n -type wagging motions. 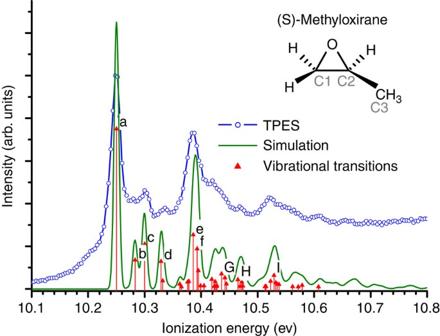Figure 1: TPES of methyloxirane HOMO band. The vibrational simulation was done at 50 K at the B3LYP/cc-pVTZ level. The size of the arrows is proportional to FC factors. The principal peaks ‘a’–‘f’ are single quantum excitations and ‘G’–‘I’ are vibrational combinations. The experimental effective resolution is 12 meV. Figure 1: TPES of methyloxirane HOMO band. The vibrational simulation was done at 50 K at the B3LYP/cc-pVTZ level. The size of the arrows is proportional to FC factors. The principal peaks ‘a’–‘f’ are single quantum excitations and ‘G’–‘I’ are vibrational combinations. The experimental effective resolution is 12 meV. Full size image PES and PECD measurements The present PECD study is based upon the analysis of Abel-inverted electron images. From the radial distribution in the total image, we obtain the PES, whereas from the LCP-RCP difference images, the dichroic parameter b 1 can be obtained, as shown in Fig. 2 . The difference images ( Fig. 2a ) readily reveal a marked vibrational structure in the radial (that is, electron energy) distribution, associated with strong forward-backward asymmetries in the angular distribution. Striking changes in the sign of the latter for some adjacent vibrational ring patterns can also be seen in the alternating colour mapping. 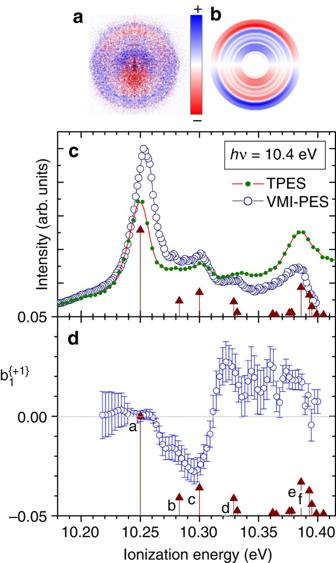Figure 2: PES and dichroic parameter at 10.4 eV for the HOMO orbital ofS-methyloxirane. (a) Raw and (b) Abel-inverted difference (LCP–RCP) parent-ion mass filtered images, obtained with the velocity map imaging (VMI) spectrometer (see text for explanation). Note that the photon beam propagates from the bottom to the top of this image. (c) VMI-PES superimposed with the reference TPES ofFig. 1. (d)curve. The sticks correspond to the calculated vibrational spectrum. The error bars were obtained by assuming a Poisson distribution of the photoelectron image pixel intensities, and then propagating the Poisson s.d. through the image inversion transformation. Figure 2: PES and dichroic parameter at 10.4 eV for the HOMO orbital of S -methyloxirane. ( a ) Raw and ( b ) Abel-inverted difference (LCP–RCP) parent-ion mass filtered images, obtained with the velocity map imaging (VMI) spectrometer (see text for explanation). Note that the photon beam propagates from the bottom to the top of this image. ( c ) VMI-PES superimposed with the reference TPES of Fig. 1 . ( d ) curve. The sticks correspond to the calculated vibrational spectrum. The error bars were obtained by assuming a Poisson distribution of the photoelectron image pixel intensities, and then propagating the Poisson s.d. through the image inversion transformation. Full size image The PES and b 1 parameter features obtained in the velocity map imaging mode at photon energy of 10.4 eV, as depicted in Fig. 2c , closely match the vibrational structure identified in the TPES. These features exhibit very distinctive and remarkable dichroic behaviour, with b 1 values ranging from a null value for peak ‘a’ to a negative value of −0.03 for ‘c’ and then switching sign within a few tens of meV to a positive ~+0.02 value for peaks ‘d’ and ‘e’. Phenomenologically, this sign change in b 1 means that the forward/backward asymmetry reverses direction for adjacent individually resolved vibrational modes. This striking behaviour of asymmetry flipping, upon vibrational (adjacent) excitation has never been observed, to our knowledge, in any molecular photoionization experiment. Moreover, this dependence of PECD with the vibrational energy content of the residual cation is completely unexpected within the usual FC assumptions and cannot be explained as a simple kinetic energy (KE) dependence as the b 1 curve is not monotonic with the KE. At this point, we effectively rule out any continuum resonance as a cause of the dramatic flip in forward/backward asymmetry. An extensive DFT calculation of the methyloxirane valence ionization continuum [23] , [24] noted no indication of shape resonances at, or below this energy. Moreover, a total ion yield spectrum of methyloxirane, as presented in Fig. 3 , shows after a marked onset located around 10.25 eV, a smooth rise until ~11 eV, corresponding to the integration of the HOMO PES peak, before rising again because of the opening of the (HOMO-1) −1 channel. No sign of any resonant feature can be seen in the spectral range corresponding to the HOMO. 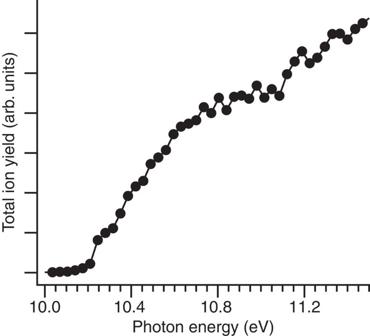Figure 3: Total ion yield spectrum of methyloxirane in the HOMO and HOMO-1 orbital region. After the ionization onset, the smooth behaviour of the ionization cross-section shows no indication of any resonant feature. The data has been normalized by the photon flux. Figure 3: Total ion yield spectrum of methyloxirane in the HOMO and HOMO-1 orbital region. After the ionization onset, the smooth behaviour of the ionization cross-section shows no indication of any resonant feature. The data has been normalized by the photon flux. Full size image As previously noted [25] , the variability of the b 1 parameter with quantum state often greatly exceeds that of the cross-section, and the PECD spectrum consequently can appear more highly resolved. One consequence of the asymmetry flipping reported here ( Fig. 2 ) is an enhanced visual demarcation of vibrational features that appear only weakly in the PES. In Fig. 4c are presented PES and PECD measurements recorded at 10.7 eV. The situation at 10.7 eV has significantly evolved within 0.3 eV, showing the strong dynamical behaviour of PECD. Here, b 1 values spread over a very large range, depending on the final vibrational energy, from −0.09 for peak ‘c’ to ~0 at higher energy. Therefore, the general KE effect is to shift b 1 towards negative values with increasing KE for all vibrational states. Most importantly, a clear non-monotonic behaviour between peaks ‘c’ and ‘d’ is superimposed again over this general trend, thus showing for both photon energies a large vibration dependence of the PECD. 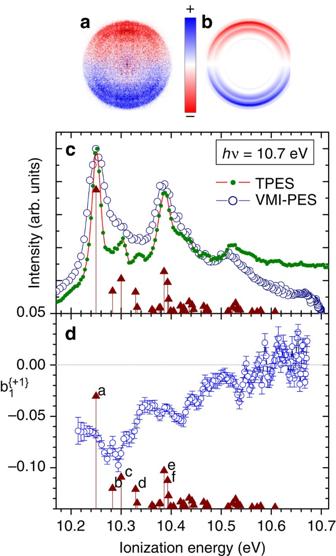Figure 4: PES and dichroic parameter at 10.7 eV for the HOMO ofS-methyloxirane. (a) Raw and (b) Abel-inverted difference (LCP–RCP) parent-ion mass filtered images obtained with the velocity map imaging (VMI) spectrometer (see text for explanation). Note that the photon beam propagates from the bottom to the top of this image. (c) VMI-PES superimposed with the reference TPES ofFig. 1. (d)curve. The sticks correspond to the calculated vibrational spectrum. The error bars were obtained by assuming a Poisson distribution of the photoelectron image pixel intensities, and then propagating the Poisson s.d. through the image inversion transformation. Figure 4: PES and dichroic parameter at 10.7 eV for the HOMO of S -methyloxirane. ( a ) Raw and ( b ) Abel-inverted difference (LCP–RCP) parent-ion mass filtered images obtained with the velocity map imaging (VMI) spectrometer (see text for explanation). Note that the photon beam propagates from the bottom to the top of this image. ( c ) VMI-PES superimposed with the reference TPES of Fig. 1 . ( d ) curve. The sticks correspond to the calculated vibrational spectrum. The error bars were obtained by assuming a Poisson distribution of the photoelectron image pixel intensities, and then propagating the Poisson s.d. through the image inversion transformation. Full size image We have observed a dramatic vibrational effect in the CPL-induced photoionization of pure randomly oriented enantiomers, well removed from any obvious resonance. Stener and co-workers first demonstrated through numerical calculations a very dramatic dependence of the predicted chiral b 1 parameter on molecular geometry [26] . In fact, the example they chose to consider was a rotation of the methyl group in methyl oxirane approximating to the torsional motion in the molecule. The variation displayed by b 1 far exceeded any corresponding dependence of the photoionization cross-section or β-parameter, although a Boltzmann average over the rotational positions returned effectively the same b 1 parameter curve as could be obtained at a fixed equilibrium geometry. We attribute this enhanced geometry dependence of b 1 to its incorporating the sine of the relative partial wave-scattering phases, these being most rapidly varying for small phase shifts differences [11] , [15] . Subsequently, combined experimental/theoretical studies have confirmed a pronounced sensitivity of the PECD effect to molecular conformation [17] , [18] , [19] , [27] , [28] . It seems plausible that this demonstrated dependence on statistical geometric structure would be somehow replicated in dynamic structural changes occasioned by vibrational motion [29] , violating the FC assumption of geometry invariant full electronic matrix elements. Vibrationally resolved measurements will be associated with a different sampling of the nuclear configuration space by the vibrational motion. This is somewhat analogous to the situation treated in vibrationally resolved circular dichroism in the angular distribution measurements on fixed-in-space CO [10] , where including integration of the electronic terms over the vibrational coordinate produces different full vibronic matrix elements for each resolved vibrational state. We can anticipate that for the randomly oriented chiral molecule photoionization, the PECD measurement will be most sensitive to this effect. This photoionization vibrational effect in PECD seems more remarkable than what has been measured in the past on fixed-in-space molecules; yet, it has been achieved without requiring molecular orientation to preserve phase information because of the intrinsically chiral nature of the targets. In contrast, non-chiral species need to be oriented in space via an extrinsic experimental chiral arrangement to preserve most of the phase information, leading, in the case of CO, to a vibration-dependent CDAD, as observed from the MF-PADs. In this context, PECD seems to offer a powerful and (for chiral species) universally applicable probe of vibrational dynamics in molecular photoionization, even from randomly oriented targets. This, of course, is the ‘natural’ situation for the ubiquitous chiral molecules in the biosphere. Such a sensitivity will be a key feature of the quickly growing field of laser-based multiphoton PECD experiments, as recently demonstrated [3] , whose outcomes may be driven by vibrational dynamics in both the intermediate and final state. In addition, our findings underline a possible importance of the temperature in the interpretation of PECD data, besides the already observed sensitivity to conformer populations. Indeed, even for a single-conformer system, the Boltzmann distribution of vibrational states in the neutral system will be projected onto the cation vibrational state, and may therefore influence measurements of the PECD asymmetry and even its absolute direction. Taking some account of this additional temperature dependence could be important for a full interpretation of PECD in, for instance, analytical contexts. This temperature dependence could also have implications in astrobiology, where PECD has been proposed as an asymmetric photon-induced process on interstellar gas-phase amino acids [2] . As PECD electron asymmetries must be mirrored by a corresponding ion recoil asymmetry, PECD could be involved in an extraterrestrial abiotic scenario linked to the origin of life’s homochirality because of its possible induction of enantiomeric excesses in a given line of sight. Molecular beam Commercial samples of S-enantiomers of methyloxirane were placed in a −17 °C-cooled reservoir, and the vapour expanded with 0.5 bar He carrier gas through a 50-μm pinhole. The supersonic expansion was skimmed to form a molecular beam and crossed at a right angle with the vacuum ultraviolet (VUV) photon beam provided by the variable polarization undulator-based beamline DESIRS [30] , at Synchrotron SOLEIL (St Aubin, France; see also http://www.synchrotron-soleil.fr/portal/page/portal/Recherche/LignesLumiere/DESIRS ). The DELICIOUS II PEPICO spectrometer In the ionization chamber, the Delicious II spectrometer [31] accelerates the produced ions and electrons in opposite directions, perpendicular to the molecular and photon beams. Briefly, this electron/ion spectrometer couples a modified velocity map imaging electron analyzer [32] with a time-of-flight ion mass spectrometer, and can be operated in electron-ion coincidence mode, used here to allowing rejection of any background electron signal not coincident with methyloxirane ions. The apparatus is capable of 5% resolving power on the edge of the detector, that is, typically 50–100 meV at 1 eV KE. In addition, Delicious II was also used in the slow electron mode [31] to record TPES with here a typical electron resolution of 10 meV. PECD data extraction The PECD at each photon energy was measured by recording several photoelectron images for alternate light helicities, and then subtracting these to obtain a difference image, which was later treated using the pBasex inversion algorithm [33] to recreate the original angular distribution of the difference. The full procedure, helicity and b 1 sign convention, as well as precautions to minimize purely instrumental effects has been described previously [25] . The DESIRS VUV beamline The DESIRS beamline delivered LCP and RCP states with corresponding Stokes parameter values of , as accurately measured by a dedicated VUV polarimeter [34] . A gas filter [35] was filled with 0.25 mbar of Argon to eliminate higher order radiation (undulator harmonics) that could be transmitted by the grating. We selected a low dispersion (200 grooves per mm), high flux grating with monochromator slit settings corresponding to a typical photon bandwidth of 7 meV at 10 eV. How to cite this article: Garcia, G. A. et al . Vibrationally induced inversion of photoelectron forward-backward asymmetry in chiral molecule photoionization by circularly polarized light. Nat. Commun. 4:2132 doi: 10.1038/ncomms3132 (2013).